Associations of autozygosity with a broad range of human phenotypes In many species, the offspring of related parents suffer reduced reproductive success, a phenomenon known as inbreeding depression. In humans, the importance of this effect has remained unclear, partly because reproduction between close relatives is both rare and frequently associated with confounding social factors. Here, using genomic inbreeding coefficients ( F ROH ) for >1.4 million individuals, we show that F ROH is significantly associated ( p < 0.0005) with apparently deleterious changes in 32 out of 100 traits analysed. These changes are associated with runs of homozygosity (ROH), but not with common variant homozygosity, suggesting that genetic variants associated with inbreeding depression are predominantly rare. The effect on fertility is striking: F ROH equivalent to the offspring of first cousins is associated with a 55% decrease [95% CI 44–66%] in the odds of having children. Finally, the effects of F ROH are confirmed within full-sibling pairs, where the variation in F ROH is independent of all environmental confounding. Given the pervasive impact of purifying selection on all populations, it is expected that genetic variants with large deleterious effects on evolutionary fitness will be both rare and recessive [1] . However, precisely because they are rare, most of these variants have yet to be identified and their recessive impact on the global burden of disease is poorly understood. This is of particular importance for the nearly one billion people living in populations where consanguineous marriages are common [2] , and the burden of genetic disease is thought to be disproportionately due to increased homozygosity of rare, recessive variants [3] , [4] , [5] . Although individual recessive variants are difficult to identify, the net directional effect of all recessive variants on phenotypes can be quantified by studying the effect of inbreeding [6] , which gives rise to autozygosity (homozygosity due to inheritance of an allele identical-by-descent). Levels of autozygosity are low in most of the cohorts with genome-wide data [7] , [8] and consequently very large samples are required to study the phenotypic impact of inbreeding [9] . Here, we meta-analyse results from 119 independent cohorts to quantify the effect of inbreeding on 45 commonly measured complex traits of biomedical or evolutionary importance, and supplement these with analysis of 55 more rarely measured traits included in UK Biobank [10] . Continuous segments of homozygous alleles, or runs of homozygosity (ROH), arise when identical-by-descent haplotypes are inherited down both sides of a family. The fraction of each autosomal genome in ROH > 1.5 Mb ( F ROH ) correlates well with pedigree-based estimates of inbreeding [11] .We estimate F ROH using standard methods and software [6] , [12] for a total of 1,401,776 individuals in 234 uniform sub-cohorts. The traits measured in each cohort vary according to original study purpose, but together cover a comprehensive range of human phenotypes (Fig. 1 , Supplementary Data 7 ). The five most frequently contributed traits (height, weight, body mass index, systolic and diastolic blood pressure) are measured in >1,000,000 individuals; a further 16 traits are measured >500,000 times. Fig. 1 Census of complex traits. Sample sizes are given for analyses of 57 representative phenotypes, arranged into 16 groups covering major organ systems and disease risk factors. HDL high-density lipoprotein, LDL low-density lipoprotein, hs-CRP high-sensitivity C-reactive protein, TNF-alpha tumour necrosis factor alpha, FEV1 forced expiratory volume in one second, FVC forced vital capacity, eGFR estimated glomerular filtration rate Full size image We find that F ROH is significantly associated with apparently deleterious changes in 32 out of 100 traits analysed. Increased F ROH is associated with reduced reproductive success (decreased number and likelihood of having children, older age at first sex and first birth, decreased number of sexual partners), as well as reduced risk-taking behaviour (alcohol intake, ever-smoked, self-reported risk taking) and increased disease risk (self-reported overall health and risk factors including grip strength and heart rate). We show that the observed effects are predominantly associated with rare (not common) variants and, for a subset of traits, differ between men and women. Finally, we introduce a within-siblings method, which confirms that social confounding of F ROH is modest for most traits. We therefore conclude that inbreeding depression influences a broad range of human phenotypes through the action of rare, recessive variants. Cohort characteristics As expected, cohorts with different demographic histories varied widely in mean F ROH . The within-cohort standard deviation of F ROH is strongly correlated with the mean (Pearson’s r = 0.82; Supplementary Fig. 3 ), and the most homozygous cohorts provide up to 100 times greater per-sample statistical power than cosmopolitan European-ancestry cohorts (Supplementary Data 5 ). To categorise cohorts, we plotted mean F ROH against F IS (Fig. 2 ). F IS measures inbreeding as reflected by non-random mating in the most recent generation, and is calculated as the mean individual departure from Hardy–Weinberg equilibrium ( F SNP ; see Methods). Cohorts with high rates of consanguinity lie near the F ROH = F IS line, since most excess SNP homozygosity is caused by ROH. In contrast, cohorts with small effective population sizes, such as the Amish and Hutterite isolates of North America, have high average F ROH , often despite avoidance of mating with known relatives, since identical-by-descent haplotypes are carried by many couples, due to a restricted number of possible ancestors. Fig. 2 Mean F ROH and F IS for 234 ROHgen sub-cohorts. Each cohort is represented by a circle whose area is proportional to the approximate statistical power ( \(N\sigma _{F_{{\mathrm{ROH}}}}^2\) ) contributed to estimates of \(\beta _{F_{{\mathrm{ROH}}}}\) . Mean F ROH can be considered as an estimate of total inbreeding relative to an unknown base generation, approximately tens of generations past. F IS measures inbreeding in the current generation, with F IS = 0 indicating random mating, F IS > 0 indicating consanguinity, and F IS < 0 inbreeding avoidance [46] . In cohorts along the y -axis, such as the Polynesians and the Anabaptist isolates, autozygosity is primarily caused by small effective population size rather than preferential consanguineous unions. In contrast, in cohorts along the dotted unity line, all excess SNP homozygosity is accounted for by ROH, as expected of consanguinity within a large effective population. A small number of cohorts along the x -axis, such as Hispanic and mixed-race groups, show excess SNP homozygosity without elevated mean F ROH , indicating population genetic structuring, caused for instance by admixture and known as the Wahlund effect. A few notable cohorts are labelled. BBJ Biobank Japan, BiB Born in Bradford, UKB UK Biobank, MESA Multiethnic Study of Atherosclerosis, TCGS Tehran Cardiometabolic Genetic Study Full size image Traits affected by F ROH To estimate the effect of inbreeding on each of the 100 phenotypes studied, trait values were regressed on F ROH within each cohort, taking account of covariates including age, sex, principal components of ancestry and, in family studies, a genomic relationship matrix (GRM) (Supplementary Data 3 ). Cross-cohort effect size estimates were then obtained by fixed-effect, inverse variance-weighted meta-analysis of the within-cohort estimates (Supplementary Data 10 ). Twenty-seven out of 79 quantitative traits and 5 out of 21 binary traits reach experiment-wise significance (0.05/100 or p < 0.0005; Fig. 3a, b ). Among these are replications of the previously reported effects on reduction in height [13] , forced expiratory lung volume in one second, cognition and education attained [6] . We find that the 32 phenotypes affected by inbreeding can be grouped into five broader categories: reproductive success, risky behaviours, cognitive ability, body size, and health. Fig. 3 Scope of inbreeding depression. a Effect of F ROH on 25 quantitative traits. To facilitate comparison between traits, effect estimates are presented in units of within-sex standard deviations. Traits shown here reached Bonferroni-corrected significance of p = 0.0005 (=0.05/100 traits). Sample sizes, within-sex standard deviations, and effect estimates in measurement units are shown in Supplementary Data 9 . FEV1 forced expiratory volume in one second. Traits are grouped by type. b Effect of F ROH on eight binary traits with associated p values. Effect estimates are reported as ln(Odds-Ratio) for the offspring of first cousins, for which E ( F ROH ) = 0.0625. Self-declared infertility is shown for information, although this trait does not reach Bonferroni corrected significant ( \({\mathrm{{OR}}}_{0.0625}\) = 2.6 ± 1.1, p = 0.0006). Numbers of cases and controls and effect estimates for all binary traits are shown in Supplementary Data 10 . c Sex-specificity of ROH effects. The effect of F ROH in men versus that in women is shown for 13 traits for which there was evidence of significant differences in the effects between sexes. For 11 of these 13 traits the magnitude of effect is greater in men than in women. Traits such as liver enzymes levels (alanine transaminase, gamma-glutamyl transferase) show sex-specific effects of opposite sign (positive in women, negative in men), which cancel out in the overall analysis. BMI body mass index, LDL low-density lipoprotein. All errors bars represent 95% confidence intervals Full size image Despite the greater individual control over reproduction in the modern era, due to contraception and fertility treatments, we find that increased F ROH has significant negative effects on five traits closely related to fertility. For example, an increase of 0.0625 in F ROH (equivalent to the difference between the offspring of first cousins and those of unrelated parents) is associated with having 0.10 fewer children [ β 0.0625 = −0.10 ± 0.03 95% confidence interval (CI), p = 1.8 × 10 −10 ]. This effect is due to increased F ROH being associated with reduced odds of having any children (OR 0.0625 = 0.65 ± 0.04, p = 1.7 × 10 −32 ) as opposed to fewer children among parents ( β 0.0625 = 0.007 ± 0.03, p = 0.66). Since autozygosity also decreases the likelihood of having children in the subset of individuals who are, or have been, married, (OR 0.0625 = 0.71 ± 0.09, p = 3.8 × 10 −8 ) it appears that the cause is a reduced ability or desire to have children, rather than reduced opportunity. Consistent with this interpretation, we observe no significant effect on the likelihood of marriage (OR 0.0625 = 0.94 ± 0.07, p = 0.12) (Fig. 3b ). All effect size, odds ratios and 95% CI are stated as the difference between F ROH = 0 and F ROH = 0.0625. The effects on fertility may be partly explained by the effect of F ROH on a second group of traits, which capture risky or addictive behaviour. Increased F ROH is associated with later age at first sex ( β 0.0625 = 0.83 ± 0.19 years, p = 5.8 × 10 −17 ) and fewer sexual partners ( β 0.0625 = −1.38 ± 0.38, p = 2.0 × 10 −12 ) but also reduced alcohol consumption ( β 0.0625 = −0.66 ± 0.12 units per week, p = 1.3 × 10 −22 ), decreased likelihood of smoking (OR 0.0625 = 0.79 ± 0.05, p = 5.9 × 10 −13 ), and a lower probability of being a self-declared risk-taker (OR 0.0625 = 0.84 ± 0.06, p = 3.4×10 −5 ) or exceeding the speed limit on a motorway ( p = 4.0 × 10 −8 ). Conservative beliefs are likely to affect these traits, and are known to be confounded with F ROH in some populations [14] , however, fitting religious participation as a covariate in UKB reduces, but does not eliminate the reported effects (Supplementary Fig. 10b , Supplementary Data 20 ). Similarly, fitting educational attainment as an additional covariate reduces 16 of 25 significant effect estimates, but actually increases 9, including age at first sex and number of children (Supplementary Fig. 10a , Supplementary Data 20 ). This is because reduced educational attainment is associated with earlier age at first sex and increased number of children, which makes it an unlikely confounder for the effects of F ROH , which are in the opposite directions. A third group of traits relates to cognitive ability. As previously reported, increased autozygosity is associated with decreased general cognitive ability, g [6] , [15] and reduced educational attainment [6] . Here, we also observe an increase in reaction time ( β 0.0625 = 11.6 ± 3.9 ms, p = 6.5 × 10 −9 ), a correlate of general cognitive ability (Fig. 3a , Supplementary Data 10 ). A fourth group relates to body size. We replicate previously reported decreases in height and forced expiratory volume [6] (Supplementary Data 21 ) and we find that increased F ROH is correlated with a reduction in weight ( β 0.0625 = 0.86 ± 0.12 kg, p = 3.4 × 10 −28 ) and an increase in the waist to hip ratio ( β 0.0625 = 0.004 ± 0.001, p = 1.4 × 10 −11 ). The remaining effects are loosely related to health and frailty; higher F ROH individuals report significantly lower overall health and slower walking pace, have reduced grip strength ( β 0.0625 = −1.24 ± 0.19 kg, p = 6.9 × 10 −24 ), accelerated self-reported facial ageing, and poorer eyesight and hearing. Increased F ROH is also associated with faster heart rate ( β 0.0625 = 0.56 ± 0.24 bpm, p = 5.9 × 10 −6 ), lower haemoglobin ( β 0.0625 = 0.81 ± 0.24 gL −1 , p = 1.6 × 10 −11 ), lymphocyte percentage, and total cholesterol ( β 0.0625 = −0.05 ± 0.015 mmol L −1 , p = 5.2 × 10 −10 ). Sex-specific effects of F ROH Intriguingly, for a minority of traits (13/100), the effect of F ROH differs between men and women (Fig. 3c , Supplementary Data 12 ). For example, men who are the offspring of first cousins have 0.10 mmol L −1 [95% CI 0.08–0.12] lower total cholesterol on average, while there is no significant effect in women; LDL shows a similar pattern. More generally, for these traits, the effect in men is often of greater magnitude than the effect in women, perhaps reflecting differing relationships between phenotype and fitness. Associations most likely caused by rare, recessive variants The use of ROH to estimate inbreeding coefficients is relatively new in inbreeding research [11] , [16] , [17] , [18] , [19] . Earlier frequency-based estimators such as F SNP and F GRM [20] , made use of excess marker homozygosity [21] , [22] , [23] and did not require physical maps. We performed both univariate and multivariate regressions to evaluate the effectiveness of F ROH against these measures. The correlations between them range from 0.13 to 0.99 and are strongest in cohorts with high average inbreeding (Supplementary Data 6 , Supplementary Fig. 6 ). Significantly, univariate regressions of traits on both F SNP and F GRM show attenuated effect estimates relative to F ROH (Supplementary Data 13 ). This attenuation is greatest in low autozygosity cohorts, suggesting that F ROH is a better estimator of excess homozygosity at the causal loci (Fig. 4c ). Fig. 4 Inbreeding depression caused by ROH. a Effect of different ROH lengths on height, compared with the effect of SNP homozygosity outside of ROH. The effects of shorter (<5 Mb) and longer (>5 Mb) ROH per unit length are similar and strongly negative, whereas the effect of homozygosity outside ROH is much weaker. The pattern is similar for other traits (Supplementary Fig. 11a ; Supplementary Data 14 ). b \({\boldsymbol{F}}_{{\mathbf{ROH}}}\) is more strongly associated than \({\boldsymbol{F}}_{{\mathbf{GRM}}}\) in a bivariate model of height. Meta-analysed effect estimates, and 95% confidence intervals, are shown for a bivariate model of height ( \({\mathrm{{Height}}}\sim F_{{\mathrm{ROH}}} + F_{{\mathrm{GRM}}}\) ). The reduction in height is more strongly associated with \(F_{{\mathrm{ROH}}}\) than \(F_{{\mathrm{GRM}}}\) , as predicted if the causal variants are in weak LD with the common SNPs used to calculate \(F_{{\mathrm{GRM}}}\) (Supplementary Note 5 ). The pattern is similar for other traits (Supplementary Fig. 15a, b ; Supplementary Data 22 ). c F ROH is a lower variance estimator of the inbreeding coefficient than F GRM . The ratio of \(\beta _{F_{{\mathrm{GRM}}}}:\beta _{F_{{\mathrm{ROH}}}}\) is plotted against \(\frac{{{\mathrm{{var}}}(F_{{\mathrm{ROH}}})}}{{{\mathrm{{var}}}(F_{{\mathrm{GRM}}})}}\) for all traits in all cohorts. When the variation of \(F_{{\mathrm{GRM}}}\) which is independent of \(F_{{\mathrm{ROH}}}\) has no effect on traits, \(\hat \beta _{F_{{\mathrm{GRM}}}}\) is downwardly biased by a factor of \(\frac{{{\mathrm{{var}}}(F_{{\mathrm{ROH}}})}}{{{\mathrm{{var}}}(F_{{\mathrm{GRM}}})}}\) (Supplementary Note 4 ). A linear maximum likelihood fit, shown in red, has a gradient consistent with unity [1.01; 95% CI 0.84–1.18], as expected when the difference between \(F_{{\mathrm{GRM}}}\) and \(F_{{\mathrm{ROH}}}\) is not informative about the excess homozygosity at causal variants (Supplementary Note 5 ). d F ROH is a better predictor of rare variant homozygosity than F GRM . The excess homozygosities of SNPs, extracted from UK Biobank imputed genotypes, were calculated at seven discrete minor allele frequencies ( \(F_{{\mathrm{MAF}}}\) ), and regressed on two estimators of inbreeding in a bivariate statistical model (see Supplementary Note 5 ). The homozygosity of common SNPs is better predicted by \(F_{{\mathrm{GRM}}}\) , but rare variant homozygosity is better predicted by \(F_{{\mathrm{ROH}}}\) . The results from real data (Fig. 4b , Supplementary Figs 15a, b and Supplementary Data 22 ) are consistent with those simulated here, if the causal variants are predominantly rare. All errors bars represent 95% confidence intervals Full size image To explore this further, we fit bivariate models with F ROH and F GRM as explanatory variables. For all 32 traits that were significant in the univariate analysis, we find that \(\widehat \beta _{F_{\mathrm{ROH}}|F_{\mathrm{GRM}}}\) is of greater magnitude than \(\widehat \beta _{F{\mathrm{GRM}}|F{\mathrm{ROH}}}\) in the conditional analysis (Fig. 4b , Supplementary Data 22 ). This suggests that inbreeding depression is predominantly caused by rare, recessive variants made homozygous in ROH, and not by the chance homozygosity of variants in strong LD with common SNPs (Fig. 4d , Supplementary Note 5 ). We also find that ROH of different lengths have similar effects per unit length (Fig. 4a , Supplementary Fig. 11a ), consistent with their having a causal effect on traits and not with confounding by socioeconomic or other factors, as shorter ROH arise from deep in the pedigree are thus less correlated with recent consanguinity. Quantifying the scope of social confounding Previous studies have highlighted the potential for F ROH to be confounded by non-genetic factors [6] , [24] . We therefore estimated the effect of F ROH within various groups, between which confounding might be expected either to differ, or not be present at all. For example, the effect of F ROH on height is consistent across seven major continental ancestry groups (Supplementary Fig. 1 , Supplementary Data 18 ), despite differing attitudes towards consanguinity, and consequently different burdens and origins of ROH. Similarly, grouping cohorts into consanguineous, more cosmopolitan, admixed and those with homozygosity due to ancient founder effects also shows consistent effects (Supplementary Fig. 2 , Supplementary Data 19 ). Equally, categorising samples into bins of increasing F ROH shows a dose-dependent response of the study traits with increased F ROH (Supplementary Data 17 and Fig. 5a, b show the response for height and ever having children; Supplementary Figs 9a–f for all significant traits). The proportionality of these effects is consistent with a genetic cause, while it is difficult to envisage a confounder proportionally associated across the entire range of observed F ROH . In particular, the highest F ROH group ( F ROH > 0.18), equivalent to the offspring of first-degree relatives, are found to be, on average, 3.4 [95% CI 2.5–4.3] cm shorter and 3.1 [95% CI 2.5–3.7] times more likely to be childless than an F ROH = 0 individual. Fig. 5 Evidence ROH effects are un-confounded. a Linear decrease in height with increasing F ROH . Average heights (in metres) is plotted in bins of increasing F ROH . The limits of each bin are shown by red dotted lines, and correspond to the offspring of increasing degree unions left-to-right. The overall estimate of \(\beta _{F_{{\mathrm{ROH}}}}\) is shown as a solid black line. Subjects with kinship equal to offspring of full-sibling or parent–child unions are significantly shorter than those of avuncular or half-sibling unions who in turn are significantly shorter than those of first-cousin unions. b Linear decrease in odds of ever having children with increasing F ROH . Linear model approximations of ln(Odds-Ratio) for ever having children (1 = parous, 0 = childless) are plotted in bins of increasing F ROH . A strong relationship is evident, extending beyond the offspring of first cousins. c ROH effects are consistent in adoptees. The ratios of effect estimates, \(\beta _{F_{{\mathrm{ROH}}}}\) , between adoptees and all individuals are presented by trait. All traits are directionally consistent and overall show a strongly significant difference from zero (average = 0.78, 95% CI 0.56–1.00, p = 2 × 10 −12 ). FEV1 forced expiratory volume in one second. d ROH effects are consistent in full siblings. The ratios of effect estimates within full siblings to effects in all individuals ( \(\beta _{F_{{\mathrm{ROH}}\_{\mathrm{wSibs}}}}:\beta _{F_{{\mathrm{ROH}}}}\) ) are presented by trait. Twenty-three of 29 estimates are directionally consistent and overall show a significant difference from zero (average = 0.78, 95% CI 0.53–1.04, p = 7 × 10 −10 ). BMI body mass index. All errors bars represent 95% confidence intervals Full size image Next, we estimated \(\beta_{{F}_{\rm{ROH}}}\) for 7153 self-declared adopted individuals in UK Biobank, whose genotype is less likely to be confounded by cultural factors associated with the relatedness of their biological parents. For all 26 significant traits measured in this cohort, effect estimates are directionally consistent with the meta-analysis and 3 (height, walking pace and hearing acuity) reach replication significance ( p < 0.004). In addition, a meta-analysis of the ratio \(\widehat \beta _{F_{{\mathrm{ROH}}\_{\mathrm{ADOPTEE}}}}:\widehat \beta _{F_{\mathrm{ROH}}}\) across all traits differs significantly from zero (Fig. 5c ; average = 0.78, 95% CI 0.56–1.00, p = 2 × 10 −12 ). Finally, the effect of F ROH was estimated in up to 118,773 individuals in sibships (full-sibling pairs, trios, etc. : \(\widehat \beta _{F_{\mathrm{ROH}\_{\mathrm{w{Sibs}}}}}\) ). F ROH differences between siblings are caused entirely by Mendelian segregation, and are thus independent of any reasonable model of confounding. The variation of F ROH among siblings is a small fraction of the population-wide variation [11] (Supplementary Data 5 ); nevertheless, 23 out of 29 estimates of \(\widehat \beta _{F_{{\mathrm{ROH}}\_{\mathrm{wSibs}}}}\) are directionally consistent with \(\widehat \beta _{F_{\mathrm{ROH}}}\) , and two (self-reported overall health and ever having children) reach replication significance. A meta-analysis of the ratio \(\widehat \beta _{F_{{\mathrm{ROH}}\_{\mathrm{wSibs}}}}:\widehat \beta _{F_{\mathrm{ROH}}}\) for all traits is significantly greater than zero (Fig. 5d ; average = 0.78, 95% CI 0.53–1.04, p = 7 × 10 −10 ), indicating a substantial fraction of these effects is genetic in origin. However, for both adoptees and siblings, the point estimates are less than one, suggesting that non-genetic factors probably contribute a small, but significant, fraction of the observed effects. Our results reveal inbreeding depression to be broad in scope, influencing both complex traits related to evolutionary fitness and others where the pattern of selection is less clear. While studies of couples show optimal fertility for those with distant kinship [25] , [26] , fewer have examined reproductive success as a function of individual inbreeding. Those that did are orders of magnitude smaller in size than the present study, suffer the attendant drawbacks of pedigree analysis, and have found mixed results [27] , [28] , [29] . Our genomic approach also reveals that in addition to socio-demographic factors and individual choice, recessive genetic effects have a significant influence on whether individuals reproduce. The discordant effects on fertility and education demonstrate that this is not just a result of genetic correlations between the two domains [30] . The effects we see on fertility might be partially mediated through a hitherto unknown effect of autozygosity on decreasing the prevalence of risk-taking behaviours. Significant effects of autozygosity are observed for self-reported risk taking, speeding on motorways, alcohol and smoking behaviour, age at first sexual intercourse and number of sexual partners. 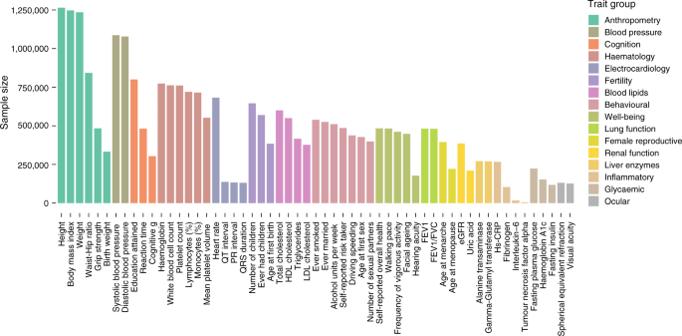Fig. 1 Census of complex traits. Sample sizes are given for analyses of 57 representative phenotypes, arranged into 16 groups covering major organ systems and disease risk factors. HDL high-density lipoprotein, LDL low-density lipoprotein, hs-CRP high-sensitivity C-reactive protein, TNF-alpha tumour necrosis factor alpha, FEV1 forced expiratory volume in one second, FVC forced vital capacity, eGFR estimated glomerular filtration rate Independent evidence for a shared genetic architecture between risk-taking and fertility traits comes from analysis of genetic correlations using LD-score regression in UKB (Supplementary Table 1 ). The core fertility traits, ever had children and number of children, are strongly genetically correlated ( r G = 0.93; p < 10 −100 ). Genetic correlations with ever-smoking and self-reported risk-taking are lower, but also significant: 0.23–0.27, p < 10 −10 . Age at first sex is strongly genetically correlated both with the fertility traits, ( r G = 0.53–0.57), and number of sexual partners, ever-smoking and risk-taking [30] ( r G = 0.42–0.60). Reproductive traits are understandable targets of natural selection, as might be walking speed, grip strength, overall health, and visual and auditory acuity. While we cannot completely exclude reverse causality, whereby a less risk-taking, more conservative, personality is associated with greater likelihood of consanguineous marriage, we note that the effects are consistent for ROH < 5 Mb, which are less confounded with mate choice, due to their more distant pedigree origins (Supplementary Fig. 11a ). This group of traits also shows similar evidence for un-confounded effects in the analysis of adoptees and full siblings (Fig. 5c, d ; Supplementary Data 16 ) and the signals remained after correcting for religious activity or education. On the other hand, for some traits that we expected to be influenced by ROH, we observed no effect. For example, birth weight is considered a key component of evolutionary fitness in mammals, and is influenced by genomic homozygosity in deer [31] ; however, no material effect is apparent here (Supplementary Data 10 ). Furthermore, in one case, ROH appear to provide a beneficial effect: increasing F ROH significantly decreases total and LDL-cholesterol in men, and may thus be cardio-protective in this regard. Our multivariate models show that homozygosity at common SNPs outside of ROH has little influence on traits, and that the effect rather comes from ROH over 1.5 Mb in length. 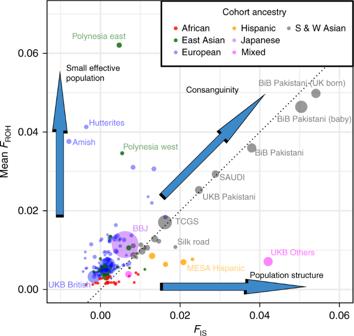Fig. 2 MeanFROHandFISfor 234 ROHgen sub-cohorts. Each cohort is represented by a circle whose area is proportional to the approximate statistical power (\(N\sigma _{F_{{\mathrm{ROH}}}}^2\)) contributed to estimates of\(\beta _{F_{{\mathrm{ROH}}}}\). MeanFROHcan be considered as an estimate of total inbreeding relative to an unknown base generation, approximately tens of generations past.FISmeasures inbreeding in the current generation, withFIS= 0 indicating random mating,FIS> 0 indicating consanguinity, andFIS< 0 inbreeding avoidance46. In cohorts along they-axis, such as the Polynesians and the Anabaptist isolates, autozygosity is primarily caused by small effective population size rather than preferential consanguineous unions. In contrast, in cohorts along the dotted unity line, all excess SNP homozygosity is accounted for by ROH, as expected of consanguinity within a large effective population. A small number of cohorts along thex-axis, such as Hispanic and mixed-race groups, show excess SNP homozygosity without elevated meanFROH, indicating population genetic structuring, caused for instance by admixture and known as the Wahlund effect. A few notable cohorts are labelled. BBJ Biobank Japan, BiB Born in Bradford, UKB UK Biobank, MESA Multiethnic Study of Atherosclerosis, TCGS Tehran Cardiometabolic Genetic Study This suggests that genetic variants causing inbreeding depression are almost entirely rare, consistent with the dominance hypothesis [1] . The alternative hypothesis of overdominance, whereby positive selection on heterozygotes has brought alleles to intermediate frequencies, would predict that more common homozygous SNPs outside long ROH would also confer an effect. The differential provides evidence in humans that rare recessive mutations underlie the quantitative effects of inbreeding depression. Previous studies have shown that associations observed between F ROH and traits do not prove a causal relationship [14] , [24] . Traditional Genome-wide Association Studies (GWAS) can infer causality because, in the absence of population structure, genetic variants (SNPs) are randomly distributed between, and within, different social groups. However, this assumption does not hold in studies of inbreeding depression, where, even within a genetically homogeneous population, social groups may have differing attitudes towards consanguinity, and therefore different average F ROH and, potentially, different average trait values. We therefore present a number of analyses that discount social confounding as a major factor in our results. Firstly, we show that the effects are consistent across diverse populations, including those where ROH burden is driven by founder effects rather than cultural practices regarding marriage. Effects are also consistent across a 20-fold range of F ROH : from low levels, likely unknown to the subject, to extremely high levels only seen in the offspring of first-degree relatives. Secondly, we show that the effects of ROH are consistent in direction and magnitude among adopted individuals, and also for short ROH which are not informative about parental relatedness. Finally, we introduce a within-siblings method, independent of all confounders, that confirms a genetic explanation for most of the observed effects. Variation in F ROH between siblings is caused entirely by random Mendelian segregation; we show that higher F ROH siblings experience poorer overall health and lower reproductive success, as well as other changes consistent with population-wide estimates. Nevertheless, average effect sizes from both adoptees and siblings are 20% smaller than population-wide estimates, confirming the importance of accounting for social confounding in future studies of human inbreeding depression. Our results reveal five large groups of phenotypes sensitive to inbreeding depression, including some known to be closely linked to evolutionary fitness, but also others where the connection is, with current knowledge, more surprising. The effects are mediated by ROH rather than homozygosity of common SNPs, causally implicating rare recessive variants rather than overdominance as the most important underlying mechanism. Identification of these recessive variants will be challenging, but analysis of regional ROH and in particular using whole-genome sequences in large cohorts with sufficient variance in autozygosity will be the first step. Founder populations or those which prefer consanguineous marriage will provide the most power to understand this fundamental phenomenon. see Supplementary Data. Overview Our initial aim was to estimate the effect of F ROH on 45 quantitative traits and to assess whether any of these effects differed significantly from zero. Previous work [7] , [11] has shown that inbreeding coefficients are low in most human populations, and that very large samples are required to reliably estimate the genetic effects of inbreeding [13] . 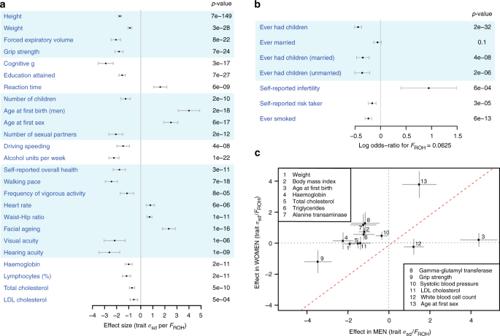Fig. 3 Scope of inbreeding depression.aEffect ofFROHon 25 quantitative traits. To facilitate comparison between traits, effect estimates are presented in units of within-sex standard deviations. Traits shown here reached Bonferroni-corrected significance ofp= 0.0005 (=0.05/100 traits). Sample sizes, within-sex standard deviations, and effect estimates in measurement units are shown in Supplementary Data9. FEV1 forced expiratory volume in one second. Traits are grouped by type.bEffect ofFROHon eight binary traits with associatedpvalues. Effect estimates are reported as ln(Odds-Ratio) for the offspring of first cousins, for whichE(FROH) = 0.0625. Self-declared infertility is shown for information, although this trait does not reach Bonferroni corrected significant (\({\mathrm{{OR}}}_{0.0625}\)= 2.6 ± 1.1,p=0.0006). Numbers of cases and controls and effect estimates for all binary traits are shown in Supplementary Data10.cSex-specificity of ROH effects. The effect ofFROHin men versus that in women is shown for 13 traits for which there was evidence of significant differences in the effects between sexes. For 11 of these 13 traits the magnitude of effect is greater in men than in women. Traits such as liver enzymes levels (alanine transaminase, gamma-glutamyl transferase) show sex-specific effects of opposite sign (positive in women, negative in men), which cancel out in the overall analysis. BMI body mass index, LDL low-density lipoprotein. All errors bars represent 95% confidence intervals To maximise sample size, a collaborative consortium (ROHgen [6] ) was established, and research groups administering cohorts with SNP chip genotyping were invited to participate. To ensure that all participants performed uniform and repeatable analyses, a semi-automated software pipeline was developed and executed locally by each research group. This software pipeline required cohorts to provide only quality-controlled genotypes (in plink binary format) and standardised phenotypes (in plain-text) and used standard software (R, PLINK [12] , [32] , KING [33] ) to perform the analyses described below. Results from each cohort were returned to the central ROHgen analysts for meta-analysis. During the initial meta-analysis, genotypes were released for >500,000 samples from the richly phenotyped UK Biobank (UKB) [10] . It was therefore decided to add a further 34 quantitative phenotypes and 21 binary traits to the ROHgen analysis. Many of these additional traits were unique to UKB, although 7 were also available in a subset of ROHgen cohorts willing to run additional analyses. In total, the effect of F ROH was tested on 100 traits and therefore experiment-wise significance was defined as 5 × 10 −4 (=0.05/100). Cohort recruitment In total, 119 independent, genetic epidemiological study cohorts were contributed to ROHgen. Of these, 118 were studies of adults and contributed multiple phenotypes, while 1 was a study of children and contributed only birth weight. To minimise any potential confounding or bias caused by within-study heterogeneity, studies were split into single-ethnicity sub-cohorts wherever applicable. Each sub-cohort was required to use only one genotyping array and be of uniform ancestry and case-status. For example, if a study contained multiple distinct ethnicities, sub-cohorts of each ancestry were created and analysed separately. At minimum, ancestry was defined on a sub-continental scale (i.e. European, African, East Asian, South Asian, West Asian, Japanese, and Hispanic were always analysed separately) but more precise separation was used when deemed necessary, for example, in cohorts with large representation of Ashkenazi Jews. In case-control studies of disease, separate sub-cohorts were created for cases and controls and phenotypes associated with disease status were not analysed in the case cohort: for example, fasting plasma glucose was not analysed in Type 2 diabetes case cohorts. Occasionally, cohorts had been genotyped on different SNP genotyping microarrays and these were also separated into sub-cohorts. There was one exception (deCODE) to the single microarray rule, where the intersection between all arrays used exceeded 150,000 SNPs. In this cohort the genotype data from all arrays was merged since the correspondence between F ROH for the individual arrays and F ROH the intersection dataset was found to be very strong ( \(\beta _{{\mathrm{merged}},{\mathrm{hap}}}\) = 0.98, r 2 = 0.98; \(\beta _{{\mathrm{merged}},{\mathrm{omni}}}\) = 0.97, r 2 =0.97). Dividing studies using these criteria yielded 234 sub-cohorts. Details of phenotypes contributed by each cohort are available in Supplementary Data 4 . Ethical approval Data from 119 independent genetic epidemiology studies were included. All subjects gave written informed consent for broad-ranging health and genetic research and all studies were approved by the relevant research ethics committees or boards. PubMed references are given for each study in Supplementary Data 2 . Genotyping All samples were genotyped on high-density (minimum 250,000 markers), genome-wide SNP microarrays supplied by Illumina or Affymetrix. Genotyping arrays with highly variable genomic coverage (such as Exome chip, Metabochip, or Immunochip) were judged unsuitable for the ROH calling algorithm and were not permitted. Imputed genotypes were also not permitted; only called genotypes in PLINK binary format were accepted. Each study applied their own GWAS quality controls before additional checks were made in the common analysis pipeline: SNPs with >3% missingness or MAF <5% were removed, as were individuals with >3% missing data. Only autosomal genotypes were used for the analyses reported here. Additional, cohort-specific, genotyping information is available in Supplementary Data 2 . Phenotyping In total, results are reported for 79 quantitative traits and 21 binary traits. These traits were chosen to represent different domains of health and reproductive success, with consideration given to presumed data availability. Many of these traits have been the subject of existing genome-wide association meta-analyses (GWAMA), and phenotype modelling, such as inclusion of relevant covariates, was copied from the relevant consortia (GIANT for anthropometry, EGG for birth weight, ICBP for blood pressures, MAGIC for glycaemic traits, CHARGE-Cognitive, -Inflammation & -Haemostasis working groups for cognitive function, CRP, fibrinogen, CHARGE-CKDgen for eGFR, CHARGE-ReproGen for ages at menarche and menopause, Blood Cell & HaemGen for haematology, GUGC for urate, RRgen, PRIMA, QRS & QT-IGC for electrocardiography, GLGC for classical lipids, CREAM for spherical equivalent refraction, Spirometa for lung function traits, and SSGAC for educational attainment and number of children ever born). Further information about individual phenotype modelling is available in Supplementary Note 1 and Supplementary Data 8 . ROH calling Runs of homozygosity (ROH) of >1.5 Mb in length were identified using published methods [6] , [11] . In summary, SNPs with minor allele frequencies below 5% were removed, before continuous ROH SNPs were identified using PLINK with the following parameters: homozyg-window-snp 50; homozyg-snp 50; homozyg-kb 1500; homozyg-gap 1000; homozyg-density 50; homozyg-window-missing 5; homozyg-window-het 1. No linkage disequilibrium pruning was performed. These parameters have been previously shown to call ROH that correspond to autozygous segments in which all SNPs (including those not present on the chip) are homozygous-by-descent, not chance arrangements of independent homozygous SNPs, and inbreeding coefficient estimates calculated by this method ( F ROH ) correlate well with pedigree-based estimates ( F PED ) [11] . Moreover, they have also been shown to be robust to array choice [6] . Calculating estimators of F For each sample, two estimates of the inbreeding coefficient ( F ) were calculated, F ROH and F SNP . We also calculated three additional measures of homozygosity: F ROH<5Mb , F ROH>5Mb and F SNP_outsideROH . F ROH is the fraction of each genome in ROH >1.5 Mb. For example, in a sample for which PLINK had identified n ROH of length l i (in Mb), i ϵ {1.. n }, then F ROH was then calculated as 
    [ F_ROH = ∑_i = 1^n l_i/3Gb ],
 (1) where F ROH<5Mb and F ROH>5Mb are the genomic fractions in ROH of length >5 Mb, and in ROH of length <5 Mb (but >1.5 Mb), respectively, and the length of the autosomal genome is estimated at 3 gigabases (Gb). It follows from this definition that 
    [ F_ROH = F_ROH > 5Mb + F_ROH < 5Mb ]. (2) Single-point inbreeding coefficients can also be estimated from individual SNP homozygosity without any reference to a genetic map. For comparison with F ROH , a method of moments estimate of inbreeding coefficient was calculated [34] , referred to here as F SNP , and implemented in PLINK by the command–het. 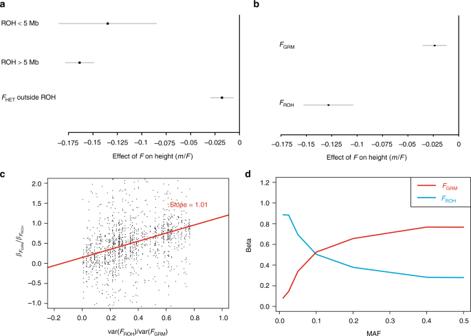Fig. 4 Inbreeding depression caused by ROH.aEffect of different ROH lengths on height, compared with the effect of SNP homozygosity outside of ROH. The effects of shorter (<5 Mb) and longer (>5 Mb) ROH per unit length are similar and strongly negative, whereas the effect of homozygosity outside ROH is much weaker. The pattern is similar for other traits (Supplementary Fig.11a; Supplementary Data14).b\({\boldsymbol{F}}_{{\mathbf{ROH}}}\)is more strongly associated than\({\boldsymbol{F}}_{{\mathbf{GRM}}}\)in a bivariate model of height. Meta-analysed effect estimates, and 95% confidence intervals, are shown for a bivariate model of height (\({\mathrm{{Height}}}\sim F_{{\mathrm{ROH}}} + F_{{\mathrm{GRM}}}\)). The reduction in height is more strongly associated with\(F_{{\mathrm{ROH}}}\)than\(F_{{\mathrm{GRM}}}\), as predicted if the causal variants are in weak LD with the common SNPs used to calculate\(F_{{\mathrm{GRM}}}\)(Supplementary Note5). The pattern is similar for other traits (Supplementary Fig.15a, b; Supplementary Data22).cFROHis a lower variance estimator of the inbreeding coefficient thanFGRM. The ratio of\(\beta _{F_{{\mathrm{GRM}}}}:\beta _{F_{{\mathrm{ROH}}}}\)is plotted against\(\frac{{{\mathrm{{var}}}(F_{{\mathrm{ROH}}})}}{{{\mathrm{{var}}}(F_{{\mathrm{GRM}}})}}\)for all traits in all cohorts. When the variation of\(F_{{\mathrm{GRM}}}\)which is independent of\(F_{{\mathrm{ROH}}}\)has no effect on traits,\(\hat \beta _{F_{{\mathrm{GRM}}}}\)is downwardly biased by a factor of\(\frac{{{\mathrm{{var}}}(F_{{\mathrm{ROH}}})}}{{{\mathrm{{var}}}(F_{{\mathrm{GRM}}})}}\)(Supplementary Note4). A linear maximum likelihood fit, shown in red, has a gradient consistent with unity [1.01; 95% CI 0.84–1.18], as expected when the difference between\(F_{{\mathrm{GRM}}}\)and\(F_{{\mathrm{ROH}}}\)is not informative about the excess homozygosity at causal variants (Supplementary Note5).dFROHis a better predictor of rare variant homozygosity thanFGRM. The excess homozygosities of SNPs, extracted from UK Biobank imputed genotypes, were calculated at seven discrete minor allele frequencies (\(F_{{\mathrm{MAF}}}\)), and regressed on two estimators of inbreeding in a bivariate statistical model (see Supplementary Note5). The homozygosity of common SNPs is better predicted by\(F_{{\mathrm{GRM}}}\), but rare variant homozygosity is better predicted by\(F_{{\mathrm{ROH}}}\). The results from real data (Fig.4b, Supplementary Figs15a, band Supplementary Data22) are consistent with those simulated here, if the causal variants are predominantly rare. All errors bars represent 95% confidence intervals [ F_SNP = O( HOM) -E( HOM)/N - E( HOM) ],
 (3) where O (HOM) is the observed number of homozygous SNPs, E (HOM) is the expected number of homozygous SNPs, i.e. \(\mathop {\sum}\nolimits_{i = 1}^N {\left( {1 - 2p_iq_i} \right)}\) , and N is the total number of non-missing genotyped SNPs. F ROH and F SNP are strongly correlated, especially in cohorts with significant inbreeding, since both are estimates of F . To clarify the conditional effects of F ROH and F SNP , an additional measure of homozygosity, F SNPoutsideROH , was calculated to describe the SNP homozygosity observed outside ROH. [ F_SNP_outsideROH = O'( HOM) - E'( HOM)/N' - E'( HOM) ],
 (4) where 
    [ O'( HOM) = O( HOM) - N_SNP_ROH ],
 (5) 
    [ E'( HOM) = ( N - N_ROH/N) ∗ E( HOM) ],
 (6) 
    N' = N - N_ROH
 (7) And N SNP_ROH is the number of homozygous SNPs found in ROH. Note that: 
    F_SNP_outsideROH≈ F_SNP - F_ROH
 (8) A further single point estimator of the inbreeding coefficient, described by Yang et al. [20] as \(\widehat F^{{\mathrm{{III}}}}\) , is implemented in PLINK by the parameter –ibc (Fhat3) and was also calculated for all samples. F_GRM = F^III = 1/N∑_i = 1^N ( x_i^2 - ( 1 + 2p_i)x_i + 2p_i^2)/2p_i( 1 - p_i),
 (9) where N is the number of SNPs, pi is the reference allele frequency of the i th SNP in the sample population and x i is the number of copies of the reference allele. Effect size estimates for quantitative traits In each cohort of n samples, for each of the quantitative traits measured in that cohort, trait values were modelled by 
    [ y = β _F_ROH∗𝐅_𝐑𝐎𝐇 + 𝐗𝐛 +ε ],
 (10) where y is a vector ( n × 1) of measured trait values, \(\beta_{{F}_{\rm{ROH}}}\) is the unknown scalar effect of F ROH on the trait, F ROH is a known vector ( n × 1) of individual F ROH , b is a vector ( m × 1) of unknown fixed covariate effects (including a mean, μ ), X in a known design matrix ( n × m ) for the fixed effects, and ε is an unknown vector ( n × 1) of residuals. The m fixed covariates included in each model were chosen with reference to the leading GWAMA consortium for that trait and are detailed in Supplementary Data 8 . For all traits, these covariates included: age (and/or year of birth), sex, and at least the first 10 principal components of the genomic relatedness matrix (GRM). Where necessary, additional adjustments were made for study site, medications, and other relevant covariates (Supplementary Data 3 ). For reasons of computational efficiency, it was decided to solve Eq. ( 10 ) in two steps. In the first step, the trait ( y ) was regressed on all fixed covariates to obtain the maximum likelihood solution of the model: 
    [ 𝐲 = 𝐗𝐛 + ε' ]. (11) All subsequent analyses were performed using the vector of trait residuals ε′ , which may be considered as the trait values corrected for all known covariates. In cohorts with a high degree of relatedness, mixed-modelling was used to correct for family structure, although, because ROH are not narrow-sense heritable, this was considered less essential than in Genome-Wide Association Studies. Equation ( 11 ) becomes 
    𝐲 = 𝐗𝐛 + 𝐮 + ε',
 (12) where u is an unknown vector ( n × 1) of polygenic effects with multivariate normal distribution of mean 0 and covariance matrix σ g 2 A , where A is the genomic relationship matrix (GRM). In these related cohorts, a GRM was calculated using PLINK v1.9 and Grammar+ residuals of Eq. ( 12 ) were estimated using GenABEL [35] . These Grammar+ residuals ( ε′ ) were used in subsequent analyses. To estimate \(\beta_{{F}_{\rm{ROH}}}\) for each trait, trait residuals were regressed on F ROH to obtain the maximum likelihood (ML) solution of the model 
    ε' = μ + β _F_ROH∗𝐅_𝐑𝐎𝐇 + ε. (13a) The sex-specific estimates of \(\beta_{{F}_{\rm{ROH}}}\) (Supplementary Data 12 ) were obtained from Eq. (13) applied to the relevant sex. For all traits, a corresponding estimates of \(\beta_{{F}_{\rm{SNP}}}\) and \(\beta_{\rm{F}_{\rm{GRM}}}\) were obtained from the models 
    ε' = μ + β _F_SNP∗𝐅_𝐒𝐍𝐏 + ε,
 (13b) 
    ε' = μ + β _F_GRM∗𝐅_𝐆𝐑𝐌 + ε
 (14) and the effects of different ROH lengths and of SNP homozygosity (Fig. 4b ) were obtained from the model 
    [ ε' = μ + ( β _1 ∗𝐅_𝐒𝐍𝐏_outsideROH) + ( β _2 ∗𝐅_𝐑𝐎𝐇 < 5𝐌𝐛);                           -62pt+ ( β _3 ∗𝐅_𝐑𝐎𝐇 > 5𝐌𝐛) + ε ]. (15) Effect size estimates for binary traits Binary traits were analysed by two methods. The primary estimates of \(\beta_{{F}_{\rm{ROH}}}\) (Fig. 3b and Supplementary Data 10 ) were obtained from full logistic models: 
    [ g( E[ 𝐲]) =𝐗𝐛 ],
 (16) where g () is the link function (logit), and where F ROH and all applicable covariates (Supplementary Datas 3 , 8 ) were fitted simultaneously. Mixed modelling for family structure was not attempted in the logistic models since an accepted method was not apparent. For all subsequent results, y was scaled by \(1/\sigma _y^2\) and analysed by linear models, as for quantitative traits, including mixed-modelling where appropriate for family studies. This method of estimating binary traits with simple linear models gives asymptotically unbiased estimates of \(\beta_{{F}_{\rm{ROH}}}\) and se( \(\beta_{{F}_{\rm{ROH}}}\) ) on the ln(Odds-Ratio) scale [36] . For all significant binary traits, a comparison of \(\widehat \beta _{F_{\mathrm{ROH}}}\) from the full model with \(\widehat \beta _{F_{\mathrm{ROH}}}\) from the linear model approximation is presented in Supplementary Fig. 8 . To give \(\widehat \beta _{F_{\mathrm{ROH}}}\) a more tangible interpretation, effect estimates are frequently quoted in the text as β 0.0625 , i.e. the estimated effect in the offspring of first cousins, where 6.25% of the genome is expected to be autozygous. Religiosity and educational attainment as additional covariates To assess the importance of potential social confounders, proxy measures of socio-economic status and religiosity were separately included in Eq. (13) as additional covariates. The modified effect estimates ( \(\widehat {\beta \prime }_{F_{\mathrm{ROH}}}\) ) were tested for significance (Supplementary Data 20 ) and compared to the uncorrected estimates ( \(\beta_{{F}_{\rm{ROH}}}\) ) (Supplementary Fig. 10a, b ). Since Educational Attainment (EA) was measured in many cohorts, this was chosen as the most suitable proxy for socio-economic status. However, since F ROH is known to affect EA directly [6] any change in \(\beta_{{F}_{\rm{ROH}}}\) when conditioning on EA cannot be assumed to be entirely due to environmental confounding. The analysis of religiosity was only carried out in UKB, where a rough proxy was available. Although no direct questions about religious beliefs were included, participants were asked about their leisure activities. In response to the question Which of the following do you attend once a week or more often? (You can select more than one) , 15.6% of UKB participants selected Religious Group from one of the seven options offered. In the models described, religiosity was coded as 1 for those who selected Religious Group and 0 for those who did not. Although this is likely to be an imperfect measure of actual religious belief it is currently the best available in a large dataset. Assortative mating Humans are known to mate assortatively for a number of traits including height and cognition [37] , and so we sought to investigate if this could influence our results, for example, by the trait extremes being more genetically similar and thus the offspring more homozygous. We see no evidence for an effect of assortative mating on autozygosity, however. Firstly, a polygenic risk score for height (see Supplementary Note 1 ), which explains 18.7% of the phenotypic variance in height, was not associated with F ROH ( p = 0.77; Supplementary Fig. 5 ). Secondly, linear relationships between traits and autozygosity extend out to very high F ROH individuals (Supplementary Figs. 9a–f ). Samples in the highest F ROH group are offspring of genetically similar parents, very likely first or second degree relatives and, for example, the height of these samples is on average 3.4 cm [95% CI 2.5–4.3] shorter than the population mean. Assortative mating would suggest this height deficit has been inherited from genetically shorter parents, but this would require an implausibly strong relationship between short stature and a propensity to marry a very close relative. Thirdly, the sex-specific effects we observe could only be explained by assortative mating if the additive heritability of these traits also differed by gender. Average trait values in groups of similar F ROH In each cohort individuals were allocated to one of ten groups of similar F ROH . The bounds of these groups were the same for all cohorts, specifically {0, 0.002, 0.0041, 0.0067, 0.0108, 0.0186, 0.0333, 0.06, 0.10, 0.18 and 1.0}. Within each group the mean trait residual ( ε′ ) and mean F ROH were calculated, along with their associated standard errors. Within each cohort the expectation of ε′ is zero at the mean F ROH , however as mean F ROH varies between cohorts (Fig. 2 , Supplementary Data 5 ) it was necessary to express ε′ relative to a common F ROH before meta-analysis. Hence, for this analysis only, the trait residuals ( ε′ ) were expressed relative to the F ROH = 0 intercept, i.e. by subtracting μ from Eq. (13). Effect of F ROH within adoptees We compared \(\beta_{{{F}_{\rm{ROH}\_{\rm{ADOPTEE}}}}}\) to cross-cohort \(\beta_{{F}_{\rm{ROH}}}\) , not that from UKB alone, as we consider the latter to be a noisy estimate of the former; estimates in UKB are consistent with those from meta-analysis. Effect of F ROH within full-sibling families In a subset of cohorts, with substantial numbers of related individuals, further analyses were performed to investigate the effect of F ROH within full-sibling families. In each of these cohorts, all second-degree, or closer, relatives were identified using KING (parameters:–related–degree 2). Full-siblings were then selected as relative pairs with genomic kinship >0.175 and IBS0 >0.001. This definition includes monozygotic twins, who were intentionally considered as part of full-sibling families. Although monozygotic twins are expected to have identical F ROH , they may not have identical trait values, and including additional trait measurements decreases the sampling error of the within-family variance estimate, hence increasing statistical power. Dizygotic twins were also included. For each individual ( j) with identified siblings, the values of F ROH and trait residual ( ε′ ) were calculated relative to their family mean (and called F j ROH_wSibs and ε j wSibs , respectively), i.e. for individual j with n full-siblings S k where k ϵ {1.. n } 
    [ F_j^ROHwSibs = F_j^ROH - 1/( n + 1)∑_iϵ{j,S_k}F_i^ROH ],
 (17) 
    [ ε _j^wSibs = ε _j^' - 1/( n + 1)∑_iϵ{j,S_k}ε' _i ]. (18) The effect of F ROH within-full-siblings ( \(\beta_{{F}_{\rm{ROH}}\_{\rm{wSibes}}}\) ) was estimated by linear regression of ε wSibs on F ROH_wSibs . Importantly, the variation of F ROH within full-siblings is entirely caused by differences in Mendelian segregation, and is therefore completely independent of all possible confounders. Hence, the effect estimates obtained by this method are estimates of the genetic effects of F ROH , unbiased by any possible confounder. Since confounding by social factors is a major concern in this field, methods that can definitively exclude this possibility are of critical importance. Between-cohort meta-analysis As is typical in genome-wide association meta-analyses (GWAMA), genetic effects were estimated within single-ethnicity sub-cohorts, and meta-analysis of the within-cohort effect sizes was used to combine results [38] . This established method eliminates any potential confounding caused by between-cohort associations between F ROH and traits. Each cohort returned estimates and standard errors of: \(\beta_{{F}_{\rm{ROH}}}\) , \(\beta_{{F}_{\rm{SNP}}},\beta_{{F}_{\rm{ROH} > {\rm{Mb}}}},\beta_{{F}_{\rm{ROH} < {\rm{Mb}}}},\beta_{{F}\_{\rm{outsideROH}}}, \beta_{{F}_{\rm{ROH}\_{\rm{wSibs}}}}\) , as well as trait means ( \(\overline {\varepsilon \prime }\) ) and standard errors within each of 10 F ROH bins. The between-cohort mean of each of these 16 estimates was then determined by fixed-effect, inverse-variance meta-analysis using the R package metafor [39] . Results shown in Figs. 3 – 5 are meta-analysed averages of the within-cohort effects. The meta-analysis was also run for various subsets of cohorts, stratified by ancestry as defined in Supplementary Data 18 . Meta-analysis estimates from these groupings are shown in Supplementary Fig. 1 . Median and 95% CI of a ratio In the analyses of adoptees (Fig. 5c ), siblings (Fig. 5d ) and potential confounders (Supplementary Figs. 10a, b ) we wished to compare the effect estimates ( \(\beta_{{F}_{\rm{ROH}}}\) ) from two different methods across a wide range of traits. The units of \(\beta_{{F}_{\rm{ROH}}}\) differ by trait so, to allow comparison across all traits, the unitless ratio of effect size estimates was calculated (for example \(\beta_{{F}_{\rm{ROH}\_{\rm{wSibs}}}}\) : \(\beta_{{F}_{\rm{ROH}}}\) ). 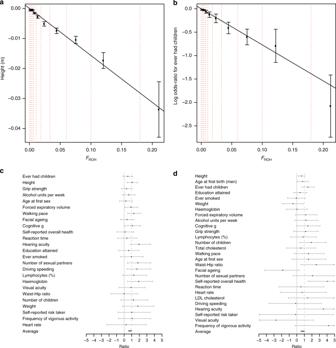Fig. 5 Evidence ROH effects are un-confounded.aLinear decrease in height with increasingFROH. Average heights (in metres) is plotted in bins of increasingFROH. The limits of each bin are shown by red dotted lines, and correspond to the offspring of increasing degree unions left-to-right. The overall estimate of\(\beta _{F_{{\mathrm{ROH}}}}\)is shown as a solid black line. Subjects with kinship equal to offspring of full-sibling or parent–child unions are significantly shorter than those of avuncular or half-sibling unions who in turn are significantly shorter than those of first-cousin unions.bLinear decrease in odds of ever having children with increasingFROH. Linear model approximations of ln(Odds-Ratio) for ever having children (1 = parous, 0 = childless) are plotted in bins of increasingFROH. A strong relationship is evident, extending beyond the offspring of first cousins.cROH effects are consistent in adoptees. The ratios of effect estimates,\(\beta _{F_{{\mathrm{ROH}}}}\), between adoptees and all individuals are presented by trait. All traits are directionally consistent and overall show a strongly significant difference from zero (average = 0.78, 95% CI 0.56–1.00,p= 2 × 10−12). FEV1 forced expiratory volume in one second.dROH effects are consistent in full siblings. The ratios of effect estimates within full siblings to effects in all individuals (\(\beta _{F_{{\mathrm{ROH}}\_{\mathrm{wSibs}}}}:\beta _{F_{{\mathrm{ROH}}}}\)) are presented by trait. Twenty-three of 29 estimates are directionally consistent and overall show a significant difference from zero (average = 0.78, 95% CI 0.53–1.04,p=7 × 10−10). BMI body mass index. All errors bars represent 95% confidence intervals Figure 5c, d and Supplementary Figs. 10a, b show the medians and 95% CI of these ratios. These were determined empirically by bootstrap since, although formulae exist for the mean and standard error of a ratio [40] , the assumption of normality is violated when \(\beta_{{F}_{\rm{ROH}}}\) /se( \(\beta_{{F}_{\rm{ROH}}}\) ) is not large. Genetic correlations in UK Biobank Genetic correlations were calculated using LD-Score Regression [41] , implemented in LDSC v1.0.0 ( https://github.com/bulik/ldsc ). Summary statistics were parsed using default parameters in the LDSC ‘munge_sumstats.py’ script, extracting only variants present in the HapMap 3 reference panel. Accuracy of F ROH measures of inbreeding effects A recent paper suggested that ROH may overestimate inbreeding effects by as much as 162% [42] ; however, this could only be the case if F ROH underestimates excess homozygosity at the causal loci by at least 162%. We do not believe this to be the case since the maximum F ROH measured in many cohorts is around 0.25 (the expectation in the offspring off first-degree relatives), and the effect size estimates from these samples are consistent with the overall estimates (Fig. 5c, d and Supplementary Fig. 9a–f ). We note that Yengo et al. applied the ROH calling parameters used here to imputed data. These parameters have been validated for called genotype data [6] but not, to our knowledge, for the higher SNP density and error rate of imputed data (see also Supplementary Note 4 ). The simple method for detecting ROH used here was well suited to our study, since it could be easily implemented on over one million samples, and most of the variation in F ROH is caused by easily-identified long ROH. [43] , [44] , [45] Reporting summary Further information on research design is available in the Nature Research Reporting Summary linked to this article.